Chimpanzees modify intentional gestures to coordinate a search for hidden food Humans routinely communicate to coordinate their activities, persisting and elaborating signals to pursue goals that cannot be accomplished individually. Communicative persistence is associated with complex cognitive skills such as intentionality, because interactants modify their communication in response to another’s understanding of their meaning. Here we show that two language-trained chimpanzees effectively use intentional gestures to coordinate with an experimentally naive human to retrieve hidden food, providing some of the most compelling evidence to date for the role of communicative flexibility in successful coordination in nonhumans. Both chimpanzees (named Panzee and Sherman) increase the rate of non-indicative gestures when the experimenter approaches the location of the hidden food. Panzee also elaborates her gestures in relation to the experimenter’s pointing, which enables her to find food more effectively than Sherman. Communicative persistence facilitates effective communication during behavioural coordination and is likely to have been important in shaping language evolution. The ability to appreciate that others have comprehension states and that these states can affect their behaviour is hypothesized to underpin the emergence of complex forms of communication in human evolution [1] , [2] , [3] . In intentional communication, the signaller has a goal and influences the comprehension state of the recipient by flexibly modifying their communication [4] , [5] , [6] , [7] . Communicative persistence is a key indicator of intentionality in humans and other primates and it precedes the transition to linguistically based communication in human infants [8] . There is growing evidence for intentionality and communicative persistence in great ape gestural signalling—defined as signalling with voluntary movements of arms, legs or bodily postures [9] , [10] , [11] . Communicative persistence can be evidenced by a signaller’s repetition or elaboration of signals in relation to different comprehension states of the recipient, until their goal is obtained, or failure is clearly indicated [8] , [12] , [13] . However, understanding communicative persistence in non-verbal animals is not straightforward; it is difficult to disentangle whether a signaller influences a recipient’s comprehension of the meaning of the signal or directly influences their behaviour (that is, makes them do something without assessing any comprehension of the signal about the goal) [5] , [14] . Studying episodes of coordination, where individuals communicate with one another in turn-taking sequences to achieve a goal that could not be accomplished individually, enables the nature and complexity of communicative persistence to be determined [15] , [16] , [17] . Communicative persistence in these contexts requires coordination of attention and communication to a task, goal and to one another, providing evidence that signallers perceive others as entities with comprehension states about the goal [18] . For instance, if persistence reflects a particular internal state, contingent upon changes in the availability of the goal itself, then only repetitions of the original signals would be expected to occur. If, on the other hand, senders are aware of the impact that their signals will have on the recipient, then they should elaborate their signalling flexibly, contingent upon the recipient’s comprehension about the goal [13] , [19] . Communicative flexibility can be examined effectively in the gestural domain because gestures are clearly directed [20] , [21] , meaningful [22] , [23] and can draw the attention of the recipient to specific spatial locations in the environment [24] . These characteristics allow the signaller’s goal in gesturing to be identified, in particular, in relation to the meaning of elaborations, and their influence on recipient responses. If communicative persistence is an unintentional expression of frustration at the goal itself, then diffuse, uninformative elaboration would be expected to occur [13] . If on the other hand, signallers perceive recipients as capable of comprehension about the goal, then they should elaborate by the use of informative signals that refer to the role of the recipient in pursuit of the desired goal, that is, inform the recipient what they want him to do [25] . For instance, when signallers direct their gestures to the recipient but fail to achieve the desired response, they may direct the recipient’s attention to a referent in the environment by the use of indicative gestures such as pointing. However, when recipients respond appropriately to the signal, signallers may use non-indicative gestures such as bobbing to affirm the recipient’s comprehension about the goal. Results from observational and experimental studies show some evidence for communicative persistence in wild and captive apes. However, these are generally restricted to less complex experimental tasks or conspecific social interactions that did not require face to face behavioural coordination from a distance through gestural signals, as in the present case, to achieve a goal [22] , [23] , [26] , [27] , [28] , [29] , [30] . For example, when presented with two food items (desirable and undesirable), in close proximity and visible during a fixed delay interval, great apes persisted with gesture production only following the (predetermined) delivery of the undesirable and not the desirable food items [6] , [31] . As the experimenter neither initiated nor responded to the apes’ communicative efforts prior to the food delivery, it is unclear whether the apes’ gestures following food delivery were in response to the experimenter’s behaviour (delivery of the undesirable food) or to the experimenter’s apparent lack of comprehension of the apes’ gestures [22] . Moreover, recent research demonstrates that when two chimpanzees were required to help each other to retrieve a desirable food reward, they relied on a relatively simple leader–follower strategy, rather than using a more elaborated form of communication to coordinate food retrieval [15] . Thus, the issue of how flexibly great apes can persist in communication to intentionally influence recipients remains unresolved [2] . In this study we examined communicative persistence in two language-trained chimpanzees, using a spatial memory task that demanded simultaneous coordination between a chimpanzee and a human interactant to find hidden food [32] , [33] , [34] , [35] . Both chimpanzees (Panzee and Sherman) recruited and directed an experimenter to search for a food item, hidden at various distances and locations, with the experimenter unaware of the location of the food. The experimenter searched by repeatedly pointing towards potential target locations, watching the chimpanzee for feedback and, based on this feedback, varying the pointing direction, pointing distance and their own distance to the target location. Both chimpanzees respond to the experimenter’s search efforts towards food by flexibly modifying their intentional gestures. Both increase the rate of non-indicative gestures when the experimenter approaches the location of the hidden food. Panzee also elaborates her gestures in relation to the experimenter’s pointing and disambiguates the experimenter’s understanding of her gestures about the location of hidden food. Panzee’s strategy enables her to find food more efficiently than Sherman. Communicative persistence facilitates effective and flexible communication and this capacity is likely to have been an important building block for language evolution. Communicative exchanges The chimpanzees used intentional gestures (for definition of intentional gestures at the level of gesture type, see Fig. 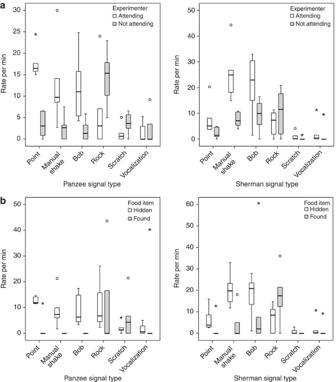Figure 1: The intentionality of chimpanzee signalling at the level of signal type. (a) Influence of experimenter visual attention towards chimpanzee on production of signals; (b) influence of object retrieval on production of signals. Intentional signalling was identified when production of signal appeared goal-directed and there was flexibility underlying usage, as evident in sensitivity to recipient’s visual attention (for example, use of auditory attention getters when recipient’s attention was directed elsewhere) and cessation of signalling when the goal has been reached6,7,8. Responses of the chimpanzees were categorized as intentional when the production was significantly higher when visual attention of the experimenter was present versus absent (visual behaviour), visual attention of the experimenter was absent versus present (auditory behaviour) and the object was hidden versus found. The tests results for each behavioural response type were the following: influence of experimenter’s visual attention: Panzee: Point (P=0.031), Manual shake (P=0.031), Bob (P=0.031), Rock (P=0.063), Scratch (P=0.063), Vocalization (P=0.5); Sherman: Point (P=0.031), Manual shake (P=0.031), Bob (P=0.031), Rock (P=0.063), Scratch (P=0.250), Vocalization (P=0.250); Influence of object hidden versus found: Panzee: Point (P=0.031), Manual shake (P=0.031), Bob (P=0.031), Rock (P=0.438), Scratch (P=0.313), Vocalization (P=1); Sherman: Point (P=0.031), Manual shake (P=0.031), Bob (P=0.031), Rock (P=0.438), Scratch (P=0.313), Vocalization (P=1). Only those behavioural response types classified as intentional were considered in further analyses. All statistical tests were performed using Wilcoxon signed-ranks test, two-tailed, with exact probabilities used,n=6 trials for each individual. Boxplots indicate medians (horizontal line in box), interquartiles (boxes) and ranges (whiskers). Stars and circles indicate outliers. 1 ) to coordinate search efforts with the experimenter (see also accompanying Supplementary Movies 1–6 of the task) and retrieve food items hidden at various distances and locations ( Table 1 ). The chimpanzees gestured only when the experimenter was visually oriented towards them ( Fig. 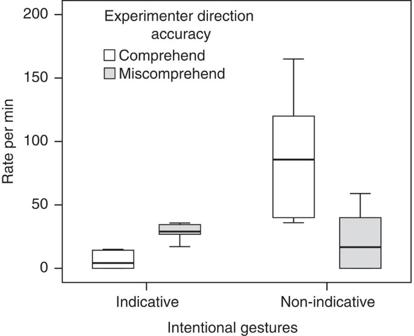Figure 2: Influence of experimenter’s comprehension of object location on Panzee’s production of indicative and non-indicative gestures. The experimenter’s comprehension of direction of object location was assessed by the accuracy of her pointing: pointing in object’s direction (comprehend), pointing in other direction (miscomprehend). Boxplots indicate medians (horizontal line in box), interquartiles (boxes) and ranges (whiskers). 1a ) and these gestures were informative, goal-directed and either indicative (for example, manual pointing) or non-indicative (manual shake and bobbing of the head or body) in terms of their ability to draw the recipient’s attention to specific spatial locations ( Table 2 ) [6] . Pointing and manual shake have been recognized as intentional gestures in previous studies [21] —in this study bobbing (which has been observed in the contexts of reunion in captive and wild chimpanzees) [20] also met the criteria of an intentional gesture ( Fig. 1 ). The experimenter and chimpanzee spontaneously influenced and shaped the directionality of each other’s behaviour by taking multiple turns in responding to indications of the location of food. On Panzee’s trials, the mean (s.d.) number of turns prior to finding the hidden food per target location was 36.3 (30.57) as compared with 43.5 (30.62) for Sherman. The majority of these turns involved intentional communication by the chimpanzees; the mean (s.d.) proportions for Panzee and Sherman were 0.76 (0.15) and 0.81 (0.06), respectively ( Table 1 ), which was significantly higher than the proportion of turns lacking intentional communication for both Panzee (Wilcoxon signed ranks test; n =6, t =0, P =0.031) and Sherman ( n =6, t =0, P =0.031). By alternating their communication in this manner, the chimpanzees and the experimenter were able to obtain the hidden food. Although the mean (s.d.) proportion of turns responded to with incorrect experimenter pointing directions was high for both Panzee (0.74 (0.18)) and Sherman (0.78 (0.17)), most trials were successful (11 out of 12) and the food item was found quickly, within a large area of woodland. The mean (s.d.) durations of trials were 2.30 (1.8) min for Panzee and 3.02 (1.5) min for Sherman. Figure 1: The intentionality of chimpanzee signalling at the level of signal type. ( a ) Influence of experimenter visual attention towards chimpanzee on production of signals; ( b ) influence of object retrieval on production of signals. Intentional signalling was identified when production of signal appeared goal-directed and there was flexibility underlying usage, as evident in sensitivity to recipient’s visual attention (for example, use of auditory attention getters when recipient’s attention was directed elsewhere) and cessation of signalling when the goal has been reached [6] , [7] , [8] . Responses of the chimpanzees were categorized as intentional when the production was significantly higher when visual attention of the experimenter was present versus absent (visual behaviour), visual attention of the experimenter was absent versus present (auditory behaviour) and the object was hidden versus found. The tests results for each behavioural response type were the following: influence of experimenter’s visual attention: Panzee: Point ( P =0.031), Manual shake ( P =0.031), Bob ( P =0.031), Rock ( P =0.063), Scratch ( P =0.063), Vocalization ( P =0.5); Sherman: Point ( P =0.031), Manual shake ( P =0.031), Bob ( P =0.031), Rock ( P =0.063), Scratch ( P =0.250), Vocalization ( P =0.250); Influence of object hidden versus found: Panzee: Point ( P =0.031), Manual shake ( P =0.031), Bob ( P =0.031), Rock ( P =0.438), Scratch ( P =0.313), Vocalization ( P =1); Sherman: Point ( P =0.031), Manual shake ( P =0.031), Bob ( P =0.031), Rock ( P =0.438), Scratch ( P =0.313), Vocalization ( P =1). Only those behavioural response types classified as intentional were considered in further analyses. All statistical tests were performed using Wilcoxon signed-ranks test, two-tailed, with exact probabilities used, n =6 trials for each individual. Boxplots indicate medians (horizontal line in box), interquartiles (boxes) and ranges (whiskers). Stars and circles indicate outliers. Full size image Table 1 Details of each trial for Panzee and Sherman. Full size table Table 2 Description of behavioural responses of Panzee and Sherman to the experimenter’s pointing gestures. Full size table Strategies of chimpanzees to lead experimenter to the food By modifying their communication in response to changes in the experimenter’s behaviour, relative to the location of the hidden food, the chimpanzees were able to successfully retrieve hidden food. The ‘common strategy’ was to modify their non-indicative gestures in relation to the experimenter’s spatial proximity to the target location. Both Panzee (Wilcoxon signed ranks test; n =6, t =0, P =0.031) and Sherman ( n =6, t =0, P =0.031) displayed a higher rate of non-indicative gestures when the experimenter was near the target location (within 0–4 m), as compared with far from the target location (>4 m). Gesturing ceased as soon as items were found by the experimenter ( Fig. 1b ), indicating that gesture production did not simply reflect high arousal in anticipation of food delivery [36] . Instead, the chimpanzees produced non-indicative gestures to provide positive feedback to the experimenter as they approached the target location, and ceased once this goal had been met. In addition to this common strategy, Panzee elaborated her gestural exchanges in relation to the accuracy of the experimenter’s pointing gestures. Panzee produced a higher rate of non-indicative gestures when the experimenter pointed toward the food rather than elsewhere (Wilcoxon signed ranks test; n =6, t =0, P =0.031, Fig. 2 ). Panzee thus shaped the experimenter’s understanding of direction by observing his directional points and giving him a ‘push’ in the right direction, at just the right moment. In contrast, incongruent experimenter responses led to a higher rate of indicative gestures. When the experimenter was far from the target location (Wilcoxon signed ranks test; n =6, t =0, P =0.031) or when their pointing was not directed toward the hidden food (Wilcoxon signed ranks test; n =6, t =0, P =0.031, Fig. 2 ), Panzee increased her pointing rate. Further, Panzee would raise her pointing hand high if the experimenter pointed too close (Wilcoxon signed ranks test; n =6, t =0, P =0.031), but lower her hand downwards when pointing was at the correct distance or beyond the target location ( n =6, t =0, P =0.031, Fig. 3 ). Panzee’s pointing gestures were directed towards the hidden object more often than elsewhere (Wilcoxon signed ranks test; n =6, t =0, P =0.031). Panzee thus used pointing to influence the experimenter’s understanding of what was ‘off track’ and what was ‘on track’, while simultaneously indicating the precise location of the hidden food. Figure 2: Influence of experimenter’s comprehension of object location on Panzee’s production of indicative and non-indicative gestures. The experimenter’s comprehension of direction of object location was assessed by the accuracy of her pointing: pointing in object’s direction (comprehend), pointing in other direction (miscomprehend). Boxplots indicate medians (horizontal line in box), interquartiles (boxes) and ranges (whiskers). 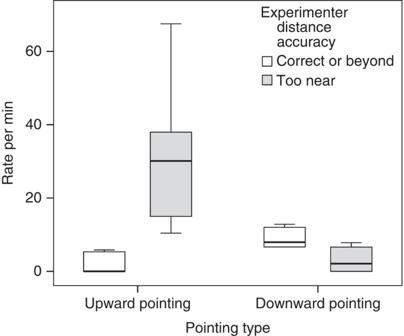Figure 3: Influence of experimenter comprehension of distance to hidden food on Panzee’s production of upward and downward pointing. The experimenter’s comprehension of distance to hidden food was assessed by the height of her pointing: pointing at correct distance or beyond object location (comprehend), pointing too near (miscomprehend). Boxplots indicate medians, interquartiles and ranges. Full size image Figure 3: Influence of experimenter comprehension of distance to hidden food on Panzee’s production of upward and downward pointing. The experimenter’s comprehension of distance to hidden food was assessed by the height of her pointing: pointing at correct distance or beyond object location (comprehend), pointing too near (miscomprehend). Boxplots indicate medians, interquartiles and ranges. Full size image In contrast, Sherman primarily responded to the overall proximity of the experimenter to the target location with manual shaking and bobbing ( Table 3 ). Panzee’s method of adjusting her gestures in relation to the accuracy of the experimenter's pointing gestures increased the efficacy of the experimenter’s search on this task [32] . There were no significant differences between the chimpanzees in terms of either experimenter or chimpanzee distance to the target at the start of the trials, or trial duration ( Table 1 ). However, the distance to the target covered by the experimenter during their search, corrected for chimpanzee communicative effort (duration of responses), was significantly greater for Panzee’s than Sherman’s trials (Mann–Whitney test, n =12, t =26, P =0.041). This shows that Panzee’s skills at communication were more efficient at directing the experimenter to the food and the success of the task was influenced by the ability of chimpanzees to communicate its location [32] . Additionally, when comparing performance by experimenters who were familiar and unfamiliar with the chimpanzees’ behaviour on this particular task, the success rate of the inexperienced experimenter was also high (5/6 trials were successful) and the trial duration did not differ between experimenters across trials matched for distance to hidden food (Mann–Whitney test, n =12, t =37, P =0.818; Table 4 ). This indicates that success was not solely determined by the experimenter’s experience on this particular task, but was instead the result of intentional communication between the chimpanzees and experimenters. Table 3 Results of statistical tests of Sherman’s responses to experimenter’s distance and pointing gestures. Full size table Table 4 Details of each trial for Panzee and Sherman with an inexperienced experimenter. Full size table The communicative flexibility reported in this paradigm [32] , [33] , [34] , [35] goes far beyond that reported in previous studies, where apes were faced with an unresponsive experimenter [6] , [31] or where conspecific social interactions did not require face to face behavioural coordination from a distance though intentional gestural signals to achieve the desired goal [20] , [22] , [23] , [26] , [27] , [28] , [29] , [30] . Here both chimpanzees dynamically and flexibly modified their intentional gestures in relation to the naive experimenter’s search efforts towards the hidden food to successfully guide the experimenter to the food item. Such communicative persistence, particularly in turn-taking episodes of communication where individuals respond communicatively to one another, is a key marker of intentional communication in humans and primates [10] , [11] , [14] . This study therefore provides some of the clearest evidence to date for such communicative persistence, and thus intentional communication, in chimpanzees. Both chimpanzees showed communicative persistence and used intentional gestural communication to guide the experimenter to a hidden food item. One interpretation could be that chimpanzees did not communicate to influence the experimenter to find hidden food, but simply adhered to the behaviour of the experimenter, allowing him to regulate the search for hidden food, while they communicated, regardless of the experimenter’s search [25] . In this case, success of chimpanzees in the current task would be due to the experimenter’s ability to read and interpret the chimpanzee’s behaviour, rather than chimpanzees’ skill at communicating. However, the success rate of the inexperienced experimenter was high, and there was no significant difference in trial duration between the experienced and inexperienced experimenters. Both experimenters were naive to the location of the food, hidden in a different location (with a varying angle and distance) on each trial, in the large woodland area. Furthermore, great care was taken to fully conceal the hiding place and, in previous experiments, uncued control objects (that are not shown to the chimpanzees) were very rarely found [32] . It is therefore clear that the search behaviour of the experimenters, and their success in finding the hidden food, was shaped by communication with the chimpanzees. Moreover, if chimpanzees simply learned the appropriate individual behaviours to get the food without perceiving the role of the experimenter in finding it, they should simply continue repeating the same movement sequences and communicative strategy, rather than modifying their behaviour in relation to the experimenter’s behaviour towards the food [25] . However, both chimpanzees used communicative means that referred to the role of the experimenter. That is, Panzee and Sherman used manual shaking and bobbing to signal that the experimenter was close to the food. Panzee also pointed higher to indicate when the experimenter’s pointing was too close or pointed lower to indicate that experimenter’s pointing was too far. This ability to make distinctions such as ‘near’ and ‘far’ is similar to some human pointing gestures [37] , and reveals sophistication comparable to the usage of some deictic words in human language. These strategies can be seen as evidence that chimpanzees understood their own and the experimenters’ actions as interdependent in finding the hidden food. The communicative strategies employed by the chimpanzees could have been shaped by the experimenter in repeated sessions of this task, or on similar tasks, ritualizing the interactions [38] . In captivity, chimpanzees can point to food locations outside their reach [39] , [40] , [41] , and some language-trained apes are more likely to use their index finger than whole hand to point, indicating that gesture use and morphology are influenced by experience [40] . However, communicative persistence more broadly is also evident in wild [20] , [22] , [23] and captive [26] , [27] , [28] , [29] chimpanzee gestural communication, indicating that the capacity is not unique to enculturated individuals. Nonetheless, in this experiment the interactive aspect of Panzee's pointing was more elaborate, producing tactics that resemble those evident in human communication [37] . By raising her arm higher when the experimenter incorrectly pointed lower, and lowering her arm when experimenter incorrectly pointed higher, Panzee may have associated her own behaviour with the experimenter’s change in pointing height. As Panzee modified her pointing in relation to changes in the height of the experimenter’s pointing relative to location of the food, and not the experimenter’s pointing height itself, the specific communicative tactics used indicate considerable flexibility in intentional communication in chimpanzees [42] . The specific and individual strategies employed in response to the experimenter’s search behaviour differed between Panzee and Sherman. Sherman’s understanding of how to use manual gestures to guide the experimenter’s search actions was more limited than Panzee's. After orienting his body toward the hidden object, he primarily responded to increases in the overall proximity of the experimenter to the target location with manual shaking and bobbing. Sherman displayed a lower frequency of points than Panzee did, and did not use or modify the morphology (height) of his pointing to indicate the location of the food. Thus, Sherman did not exploit the communicative potential of pointing as fully as Panzee did to guide the experimenter’s understanding in this task. While Sherman’s behaviour indicates that he was sensitive to the experimenter’s behaviour in relation to the food location, Panzee appears to have understood the experimenter’s comprehension of her communicative gestures about the location of the hidden food. By tailoring her communicative signals to accommodate the experimenter’s level of comprehension, Panzee was significantly more effective than Sherman at directing the experimenter to the food. The different strategies used by Panzee and Sherman reveal the importance of intentional communication in effectively coordinating behaviour [13] . Both Panzee and Sherman responded to the experimenter’s overall proximity to the target location. Panzee also responded to the experimenter’s understanding of her gestures, by confirming accurate searches and correcting inaccurate searches. When the experimenter pointed to different referents in the environment, Panzee agreed or disagreed with the experimenter’s interpretation and was able to retrieve the food items more efficiently than Sherman, showing that intentional communication can increase the efficiency of attaining goals. The capacity for chimpanzees to intentionally coordinate to obtain desired goals appears to be more sophisticated than previously demonstrated, and this level of skilled communication probably would have been present in early humans. It is likely to be a component of the general cognitive and communicative capacities that underpinned the evolution of language. In one scenario for the evolution of language, selection for enhanced communication took place in the context of coordinating social foraging [3] , [43] , [44] , [45] . The communicative strategies employed by chimpanzees in our study suggest that intentionally coordinating to obtain desired goals may have been an important aspect of social behaviour and foraging in early humans. By reformulating the understanding of the location of the resource by communicative signals, and confirming and disconfirming this understanding, two or more interactants would have increased their efficiency in foraging, hunting or other joint activities. In the absence of language, gesturing (with arm, hand, head, or whole body) to different referents in the environment may have acted as a translation of another’s intentions into communicative signals, facilitating the mapping between communicative signals and real world events. The use of nonverbal signals such as hand signals to coordinate joint activities in hunter–gatherer groups can potentially provide insights into this process, as the hunter–gatherer lifestyle was dominant during the majority of human evolution [46] . When hunting, many different hunter–gatherer groups use an extensive range of hand signals to coordinate joint activity—these include Congo Pygmies [47] , Aboriginal Australians [48] and two Kalahari Khoe-speaking groups [49] . Further, a cross-cultural comparison of hunter–gatherer groups demonstrated that hand signals occur more frequently in societies that have a higher dependence on hunting for subsistence [50] . The use of hand signals thus appears to be important in coordinating joint activities across groups of hunter–gatherers. The context of joint activity may have provided an arena for the acquisition of linguistically based communication from learnt, ritualized signals in our hominin ancestors [3] . The intentionality in gestural communication might indicate that language evolution occurred partially in the gestural domain [9] . Gestures frequently co-occur with vocalizations; however, whereas gestures can intentionally convey meaning to recipients, vocalizations seem to be unintentional from the signaller’s perspective [5] , [20] , [21] , [22] , [23] . The scaffolding of vocalizations by intentional gestures may have enabled the attribution of meaning to vocalizations and a gradual move towards intentional communication in the vocal domain [21] , [51] , [52] . Although whether such a gestural stage was necessary is a matter of debate [27] , [53] , studying processes of vocal and gestural intentional communication in both humans and non-human primates in the context of coordinating joint activity may provide important insights into language evolution [26] , [27] , [28] . Subjects The subjects were two chimpanzees ( Pan troglodytes ) — Panzee (female, 19 years old) and Sherman (male, 31 years old) at Georgia State University's Language Research Center. Both chimpanzees had been reared from an early age by human caregivers and given extensive exposure to lexigrams, which they use in everyday interactions with humans [33] , [51] , [54] . Both chimpanzees had been involved in cognitive research in topics such as language acquisition, long-term memory and numerical competence [55] , [56] . The data for the current task have been collected during 2005 and 2007 to examine recall memory, performance in simulated foraging problems and use of the lexigram keyboard [32] , [33] , [35] , but the communication strategies used have not previously been systematically examined through video analysis. These research methods were approved by the Institutional Animal Care and Use Committee of Georgia State University. Environment and apparatus Panzee and Sherman were housed in indoor and outdoor enclosures connected by a 1-m long tunnel. The indoor enclosure was visually isolated from both the outdoor enclosure and the area surrounding the outdoor enclosure. The test objects were concealed in an area of woodland measuring ~350 m 2 adjacent to the outdoor enclosure. The chimpanzees were provisioned with fruits, vegetables, chow, grains and nuts and were not food-deprived during trials. The indoor and outdoor enclosures each contained a lexigram keyboard, with a total of 256 different lexigrams per board [32] , [33] , [35] . Design and procedure Each chimpanzee was tested individually in the outdoor enclosure, taking part in six trials. In each trial, Experimenter 1 hid a food item 3–26 m from the outdoor enclosure under natural cover (for example, log, soil, leaves, branches) in a trial-unique location in the surrounding woodland, while the chimpanzee was watching ( Table 1 ), concealing any signs of hiding place (for example, breaking up of soil). The chimpanzee could not enter the woodland itself. In order to retrieve the food, the chimpanzee had to recruit the assistance of an uninformed person (Experimenter 2) and direct him to the food item. Experimenter 2 was a keeper, familiar to the chimpanzees, and experienced in conducting the experiment. Additionally, three trials for each chimpanzee were conducted with a keeper familiar to the chimpanzees but naive to this experimental task. Two different camera operators filmed food hiding and food retrieval parts of the experiment. Food retrieval was filmed by the camera operator, who was in full view of the experimenter and was unaware where the object was hidden. Experimenter 2 started near the outdoor enclosure and watched for the chimpanzee’s initial directional gesture, then walked in that direction, and stopped to take further directions. Experimenter 2 also would face and ‘query’ the chimpanzee periodically by pointing (with a 1.5-m long stick) in various directions of possible travel, by noting which of these directions evoked immediate bobbing/shaking responses by the chimpanzee (rather than continued pointing), and by moving further in that direction, iterating the process. If the food was found, it was offered to the chimpanzee. During the trials, both the chimpanzee’s and the experimenter’s behaviour were videotaped. Chimpanzee behaviour Behavioural responses of the chimpanzee to the experimenter’s pointing gestures were coded. A response started immediately after the pointing gesture of the experimenter was made and ended when the experimenter made another pointing gesture, started walking or searched through the groundcover with the stick. Indicative gestures made by the chimpanzees that were coded included any movement that appeared to be aimed at a specific distal target or a lexigram keyboard, using both an extended index finger and open hand. The morphology of indicative gestures towards the hidden object was described in terms of the arm, forearm and finger positions and classified as follows: indicate up (arm, forearm and finger directed vertically up) or indicate down (arm, forearm and finger directed horizontally or down). Additionally, the direction of gesturing was recorded using the following categories: object (pointing in the direction of the object), other direction. Non-indicative gestures coded included armshake, defined as any shaking or swinging of one or both hands or arms repeatedly; bobbing (subject bobs and weaves with head or whole body in bowing position upwards or forwards) and rocking (subject stands or sits and rocks its body from side to side or from forwards to backwards). Two additional behavioural responses recorded were scratching and vocalizations (for full descriptions of categories coded see Table 2 ). Experimenter behaviour The trial started when Experimenter 2 arrived outdoors and began to interact with the chimpanzee (as opposed to when they interacted indoors), and the end of the trial was the moment the food item was found, removed from its location and given to the chimpanzee. The experimenter’s search behaviour (pointing with the stick) was recorded when the experimenter was standing in one place. All potential pointing gestures made by the experimenter while walking were excluded because they were not responded to by the chimpanzees and it was not always possible to reliably determine the accuracy of these pointing gestures relative to the food location. Each time the experimenter made a pointing gesture, the following three pieces of information were recorded. First, the distance of the experimenter to the hidden object, determined from a map of the area of woodland and the number of steps taken by the experimenter, was categorized as close (0–4 m between experimenter and the object) or far (>4 m). Second, the direction of the experimenter’s pointing gestures was coded as follows: point towards the object (experimenter pointing in the direction of a hidden object, the location of which is within the experimenter’s field of vision) or point elsewhere (experimenter pointing in a direction other than towards the hidden object). Third, the experimenter’s accuracy at indicating distance to the object was recorded, as evidenced by the height at which the experimenter held the end of pointing stick relative to the object’s location. This was scored as correct, too far or too close, by assessing whether hidden object fell inside, outside or on the circle visually drawn by the end of line extended from the end of the stick held by the experimenter. Finally, the visual attention of the experimenter to the chimpanzee was recorded as attention present (experimenter looking at the chimpanzee, as judged from the direction of his head) or absent (any other direction). The presence of the object was coded as object absent (object hidden) or object found (object located and removed from the hiding place by the experimenter); for these analyses, the behavioural responses of the chimpanzees were recorded when the experimenter was either locomoting or standing and pointing in a direction or inspecting the surface of the ground. The coding of the responses ended when the experimenter disengaged from the chimpanzee and left the area. Analyses For the main analyses of chimpanzee behaviour during trials with the experienced experimenter, each subject was analysed individually. For each subject, data from all six trials were pooled for analyses, with paired comparisons used to analyse behaviour patterns. As trials varied in length, all behaviours were either converted to rates per min or proportions of all points. Distance per min of response was calculated by dividing the distance of the experimenter from the target at the beginning of the trial by the total chimpanzee response duration to the experimenter’s pointing gestures during that trial. The additional trials with an inexperienced experimenter, to examine whether experience of the experimenter affected the success in finding food, were pooled for both chimpanzees, matching trials in terms of the chimpanzee taking part in the trial and the distance to the food hidden. Non-parametric statistics were used with the alpha level set at 0.05 and all tests were two-tailed. One trial for each chimpanzee was coded by a second observer and agreement (Cohen’s Kappa) was good to excellent for both experimenter and chimpanzee behaviour ranging from 0.71 to 0.83. How to cite this article: Roberts, A.I. et al . Chimpanzees modify intentional gestures to coordinate a search for hidden food. Nat. Commun. 5:3088 doi: 10.1038/ncomms4088 (2014).